Probing molecule-like isolated octahedra via phase stabilization of zero-dimensional cesium lead halide nanocrystals Zero-dimensional (0D) inorganic perovskites have recently emerged as an interesting class of material owing to their intrinsic Pb 2+ emission, polaron formation, and large exciton binding energy. They have a unique quantum-confined structure, originating from the complete isolation of octahedra exhibiting single-molecule behavior. Herein, we probe the optical behavior of single-molecule-like isolated octahedra in 0D Cesium lead halide (Cs 4 PbX 6 , X = Cl, Br/Cl, Br) nanocrystals through isovalent manganese doping at lead sites. The incorporation of manganese induced phase stabilization of 0D Cs 4 PbX 6 over CsPbX 3 by lowering the symmetry of PbX 6 via enhanced octahedral distortion. This approach enables the synthesis of CsPbX 3 free Cs 4 PbX 6 nanocrystals. A high photoluminescence quantum yield for manganese emission was obtained in colloidal (29%) and solid (21%, powder) forms. These performances can be attributed to structure-induced confinement effects, which enhance the energy transfer from localized host exciton states to Mn 2+ dopant within the isolated octahedra. Over the past few years, inorganic lead halide perovskites have attracted great attention as a promising optoelectronic material for light-emitting devices, photodetectors, and low-threshold lasers, owing to their high photoluminescence quantum yield (PL QY), narrow emission, and tunable band gap [1] , [2] , [3] , [4] . The basic building block in these material is PbX 6 octahedra (where X is a halogen), whose diverse connectivity can produce structures with various dimensionalities, ranging from three-dimensional (3D) to zero-dimensional (0D) [5] , [6] , [7] . The 3D inorganic perovskites, with general formula APbX 3 (A = Cs, Rb, and X = Cl, Br, or I), consist of an extended network of corner-sharing PbX 6 octahedra with cavities occupied by A ions [8] , [9] . Despite being the most explored material, the poor chemical stability of 3D perovskites against moisture, inherent phase transformation, and ion migration make their low-dimensional counterparts more favorable for optoelectronic applications [4] , [6] , [10] . In particular, 0D inorganic perovskite-like Cs 4 PbX 6 system have crystal structure in which the PbX 6 octahedra are decoupled from each other by the surrounding Cs + ions. The complete isolation of octahedra leads to strong quantum confinement and exciton–phonon interactions, which in turn can result in exciton localization, self-trapping, and polaron formation [10] . The optical features of 0D Cs 4 PbX 6 are governed by transitions between the electronic states of Pb 2+ ions, and its broad ultraviolet (UV) emission has been assigned to the radiative decay of Frenkel excitons at Pb 2+ sites [11] , [12] , [13] , [14] , [15] . However, the origin of their PL in the visible range is still under debate because of mixed views on the efficient green luminescence (QY of 45%) of Cs 4 PbBr 6 , which some studies have been attributed to the minor 3D CsPbBr 3 nanoscale impurity [3] , [16] , [17] , [18] . Nikl et al. [12] reported a UV emission band at 355 nm for Cs 4 PbCl 6 single crystals, assigning to Pb 2+ ion emission, originating from the optical transitions of 3 P 0 , 1 → 1 S 0 in the isolated PbCl 6 octahedra, similar to Pb 2+ doping in the alkali halide hosts [12] . In addition, the coexistence of 3D CsPbCl 3 -like impurity was noted by 414 nm emission in Cs 4 PbCl 6 . While, Mohammed’s group [19] reported Cs 4 PbBr 6 characteristic with two broad UV emissions at 340 nm (high-energy) and 400 nm (low-energy) attributing to Pb 2+ ion and charge-transfer band denoted as “D-state”, respectively. D-state emission originates via the transfer of excited electrons from (PbBr 6 ) 4 – octahedra to the Pb 2+ occupying Cs sites (D-states), through their strong coupling in Cs 4 PbX 6 host [19] . Therefore, 0D Cs 4 PbX 6 behave as an ideal host–guest system, with periodically doped individual PbX 6 species in a wide band gap matrix. However, though many reports attribute the green emission (512 nm) to the intrinsic property of Cs 4 PbBr 6, we believe it arise from the coexistence of CsPbBr 3 impurity, similar to 414 nm emission of Cs 4 PbCl 6 [12] . Nevertheless, 0D cesium lead halide perovskites still represent largely unexplored and intriguing perovskite-like material, expected to exhibit interesting optoelectronic properties, due to their strongly localized excitons and high exciton binding energies (150 to 380 meV) [3] , [20] , [21] . The coexistence of 3D CsPbX 3 impurity has precluded a detailed understanding on the optical properties of Cs 4 PbX 6 , leading to a growing demand for their synthesis in pure form and their phase stabilization. Solvent washing has been recently reported for the synthesis of Cs 4 PbBr 6 free from CsPbX 3 impurity, which, however, is inadequate to treat the chloride compositions due to their poor solubility [3] . As the inevitable coexistence of CsPbX 3 phase represents a major drawback, new synthetic strategies are of utmost interest for obtaining pure Cs 4 PbX 6 nanocrystals with reduced CsPbX 3 impurity. Recently, the molecule-like behavior of Cs 4 PbBr 6 has been discussed in terms of charge carrier transport and polaron formation, arising from weak interactions between isolated octahedra [10] . Thus, understanding the fundamental optoelectronic behavior of 0D Cs 4 PbX 6 would promote the development of bulk perovskite-based devices. Incorporation of transition metal ions such as manganese (Mn 2+ ) in the semiconductor nanocrystal leads to interesting optoelectronic properties by modulating the electronic properties of the host, providing new routes for designing solid-state lighting and light-harvesting devices [22] , [23] . Hence, Mn 2+ ions can serve as the sensitive probe for investigating the local structure of the host and altering its optical and electronic behavior. Thus far, the potential effect of isovalent cation doping on the isolated octahedral units of Cs 4 PbX 6 remains unexplored, particularly in terms of phase stabilization and optical properties. In this work, we probe the optical behavior of isolated octahedra in the Cs 4 PbX 6 (X = Br, Cl, Br/Cl) by introducing Mn 2+ at the octahedral sites and explore its phase stabilization over commonly coexisting CsPbX 3 impurity. The luminescence measurements show that Mn 2+ dopant significantly alter the optical properties of different host emissive states in the Cs 4 PbX 6 . The dopant emission is controlled by adjusting the band gap of Cs 4 PbX 6 through halide identity, facilitating energy transfer for enhancing the dopant emission efficiency in both colloidal and solid forms. The quantum-confined structure of 0D Cs 4 PbX 6 further improves the stability of the host and efficiency of the dopant emission, particularly in their solid form. 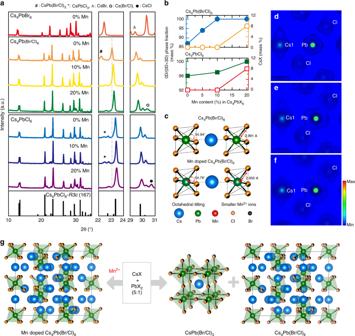Fig. 1 Local and bulk structures of Mn2+-doped Cs4PbX6.aX-ray diffraction patterns of Mn2+-doped Cs4PbX6series with different doping concentrations showing the rhombohedral structure is preserved after Mn-doping. Selected 2θrange of (22 to 24° and 29 to 31°) XRD patterns were presented. A monotonic shift of the XRD peak at Bragg’s angle at 23.4° towards higher 2θis the result of progressive lattice contraction as the Mn2+concentration increases, due to the substitutional replacement of Pb2+with isovalent but smaller Mn2+ions. The additional impurity cubic phases of 3D CsPb(Br/Cl)3, 3D CsPbCl3, CsBr, Cs(Br/Cl), and CsCl were denoted as hash, asterisk, triangle, open circle, and closed circle, respectively. It is to be noted that the Cs:Pb precursor ratio was fixed at 5:1 for all the samples of Cs4PbX6(Br, Cl, and Br/Cl).bPhase fraction of the desired 0D Cs4PbX6perovskite with respect to 3D CsPbX3perovskite phase and segregation of CsX, with varying Mn concentration in the Cs4PbX6synthesis.cOctahedral tilting/distortion without and with Mn doping (10% Mn) causing the phase stabilization of Cs4Pb(Br/Cl)6structure. Electron density distribution profile derived from Maximum Entropy method for thedundoped Cs4PbCl6,eCs4PbCl6:10% Mn, andfCs4PbCl6:20% Mn, along the (010) plane.gSchematic representation of phase stabilization of Cs4PbX6perovskite structure upon Mn2+incorporation Mn 2+ -doped Cs 4 PbX 6 nanocrystals A series of 0D Cs 4 PbX 6 (X = Br, Br/Cl, and Cl) nanocrystals, doped with manganese, were synthesized via modified reverse microemulsion method (Supplementary Figure 1 and Supplementary Note 1 ) [20] . A short-chain alkylamine (octylamine) surfactant was employed instead of the previously reported long-chain oleylamine to control size and morphology [20] . The exact composition of the synthesized undoped and Mn 2+ -doped Cs 4 Pb(Br/Cl) 6 (denoted as mixed halide) analogs are Cs 4 PbBr 2 Cl 4 and Cs 4 Pb 1 – x Mn x Br 2–2 x Cl 4+2 x , respectively, with x varying from 0.05 (5% Mn) to 0.80 (80% Mn). The Pb/Mn ratios were estimated from inductively coupled plasma−optical emission spectroscopy (Supplementary Table 1 ). For simplicity, the synthesized samples were represented as Cs 4 PbX 6 : x % Mn, where X = (Br/Cl), Cl, and Br; and x = percentage of Mn concentration with respect to displaced lead ions. Local and bulk structure The crystal structure of Cs 4 PbX 6 consists of caged PbX 6 octahedra, isolated by interspersed Cs–X bridges [21] . Two types of Cs sites are present: the Cs(1) site form an alternating octahedra with PbX 6 , whereas the Cs(2) trigonal prisms share one triangular face to form infinite [CsPbX 6 ] n 3 – chains along the [001] direction [24] . The synthesized samples were highly crystalline matching with the rhombohedral Cs 4 PbX 6 phase (X = Br, Br/Cl, and Cl; space group: R \(\bar 3\) c ) as presented in Fig. 1a . However, in the undoped Cs 4 PbX 6 , the presence of 3D CsPbX 3 impurity were clearly apparent in all the halide analogs (Fig. 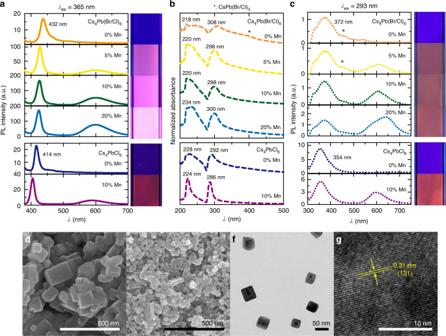Fig. 2 Luminescent properties of Mn2+-doped Cs4PbX6.aPL spectra of Mn2+-doped Cs4PbX6colloids were measured under 365 nm excitation, where X = Br/Cl and Cl, with Mn contents denoted as 0% Mn, 5% Mn, 10% Mn, and 20% Mn and the insets shows the respective samples under 365 nm UV lamp.bUV-Vis spectra of Mn2+-doped Cs4PbX6colloids.cPL spectra of Mn2+-doped Cs4PbX6colloids were measured under 290 nm excitation and the insets shows the respective samples under 254 nm UV lamp. The PL spectra presented are the PL intensities corrected using optical density. The asterix mark denote the 3D CsPb(Br/Cl)3phases. FE-SEM images ofdundoped Cs4Pb(Br/Cl)6andeCs4Pb(Br/Cl)6:10% Mn, andf,gHR-TEM images of Cs4Pb(Br/Cl)6:10% Mn. A lattice spacing of 0.31 nm corresponding to (131) plane of rhombohedral structure of Cs4Pb(Br/Cl)6 1a , Supplementary Figure 2 , and Supplementary Note 2 ). Despite using high Cesium content (Cs:Pb = 5:1), formation of undesired CsPbX 3 phase were observed in the undoped Cs 4 PbX 6 probably due to localized occurrence of Cs-deficient regions. Fig. 1 Local and bulk structures of Mn 2+ -doped Cs 4 PbX 6 . a X-ray diffraction patterns of Mn 2+ -doped Cs 4 PbX 6 series with different doping concentrations showing the rhombohedral structure is preserved after Mn-doping. Selected 2 θ range of (22 to 24° and 29 to 31°) XRD patterns were presented. A monotonic shift of the XRD peak at Bragg’s angle at 23.4° towards higher 2 θ is the result of progressive lattice contraction as the Mn 2+ concentration increases, due to the substitutional replacement of Pb 2+ with isovalent but smaller Mn 2+ ions. The additional impurity cubic phases of 3D CsPb(Br/Cl) 3 , 3D CsPbCl 3 , CsBr, Cs(Br/Cl), and CsCl were denoted as hash, asterisk, triangle, open circle, and closed circle, respectively. It is to be noted that the Cs:Pb precursor ratio was fixed at 5:1 for all the samples of Cs 4 PbX 6 (Br, Cl, and Br/Cl). b Phase fraction of the desired 0D Cs 4 PbX 6 perovskite with respect to 3D CsPbX 3 perovskite phase and segregation of CsX, with varying Mn concentration in the Cs 4 PbX 6 synthesis. c Octahedral tilting/distortion without and with Mn doping (10% Mn) causing the phase stabilization of Cs 4 Pb(Br/Cl) 6 structure. Electron density distribution profile derived from Maximum Entropy method for the d undoped Cs 4 PbCl 6 , e Cs 4 PbCl 6 :10% Mn, and f Cs 4 PbCl 6 :20% Mn, along the (010) plane. g Schematic representation of phase stabilization of Cs 4 PbX 6 perovskite structure upon Mn 2+ incorporation Full size image Upon Mn incorporation, the Bragg’s peak at 23° monotonically shifts to higher 2 θ , suggesting the substitution of Pb 2+ with smaller Mn 2+ ion in Cs 4 PbX 6 (X = Br, Br/Cl, Cl), which is also evidenced from the decrease in lattice parameters (Table 1 , Supplementary Tables 2 to 4 ) [24] , [25] . Lattice contraction of 0.3% and volume change of 2%, after Mn (20% Mn) doping, resulted in the shortening of lead halide (Pb–Br/Cl) bond lengths and similar feature was also noted in chloride analog (Supplementary Table 5 , 6 ). The strong bonding nature upon Mn doping is evidenced from high bond-dissociation energy of Mn–Cl (361 kJ mol −1 ) than Pb–Br bonds (247 kJ mol −1 ) [26] . 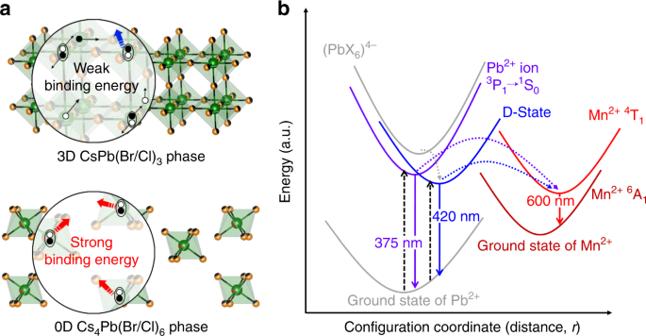Fig. 5 Mechanism of energy transfer from host states to Mn2+.aIllustration of high exciton binding energy (at above 150 meV) due to the localized excitons formed in the isolated octahedra of 0D Cs4PbX6(X = Cl, Br/Cl) perovskite, compared to low binding energies (less than 60 meV) of 3D CsPbX3perovskite, where filled and hollow circles represent electrons and holes, respectively.bConfigurational coordinate representation of Cs4Pb(Br/Cl)6perovskite depicting Pb2+-based (3P0,1→1S0transition) and D-state emissions, and their energy transfer to the Mn2+energy levels. The long dash and dotted arrows depicts the excitation and energy transfer process leading to emission (solid arrows) The valence states and substitution of Mn 2+ ions at the isolated octahedral PbX 6 sites was reaffirmed from X-ray photoelectron spectroscopy and electron spin resonance results, respectively (Supplementary Figures 3a to 3f and Supplementary Note 3 ) [22] , [27] , [28] . Quantification of multiple crystalline phases (Cs 4 PbX 6 and CsPbX 3 ) in the synthesized samples were estimated using Rietveld refinement of X-ray diffraction (XRD) results. Interestingly, Mn doping resulted in a decrease in the phase fraction (mass%) of 3D CsPbX 3 impurity, which further reduced with Mn content in both Br/Cl and Cl analogs, as shown in Fig. 1b . In other words, the phase fraction of 0D Cs 4 Pb(Br/Cl) 6 with respect to the total (0D+3D) phase gradually increased from 86 to 100% upon increasing Mn concentration from 0 to 20%. This increase in the phase fraction of Cs 4 PbX 6 was also apparent in the pure chloride and bromide analog (Supplementary Figure 2 ), suggesting that Mn 2+ incorporation in the framework favors the formation of Cs 4 PbX 6 phase, while preventing the undesirable CsPbX 3 phase. A CsPbX 3 impurity-free Cs 4 Pb(Br/Cl) 6 phase was obtained with 10% Mn content. Despite the complete suppression of CsPbX 3 , additional CsX (8%) phase tends to precipitate at higher Mn (above 10% Mn) content in both Cs 4 Pb(Br/Cl) 6 and Cs 4 PbCl 6 (Fig. 1b ). Since the presence of Mn 2+ in the lattice favors the Cs 4 PbX 6 formation, the excess Cs precursor (5:1) which is used to favor the 0D phase, tend to segregate as CsX at higher Mn concentration. 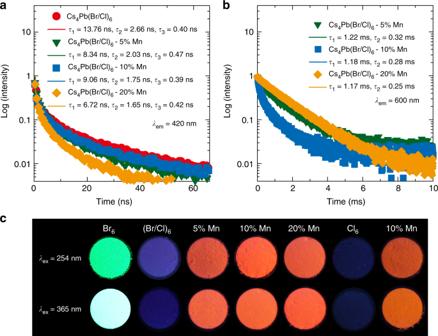The CsX formation could be further prevented by decreasing the Cs precursor (Cs:Pb = 4.5:1) in the Mn 2+ -substituted samples, leading to pure Cs 4 PbX 6 nanocrystals (Supplementary Figure 4 ). Fig. 4 Lifetime of Mn2+-doped Cs4PbX6. Time-resolved PL spectra of Cs4Pb(Br/Cl)6colloids excited at 375 nm and monitoring the D-state and Mn2+emission ata420 andb600 nm, respectively.cImages of Cs4PbX6perovskite solids under 254 and 365 nm UV lamp, which are denoted by their respective halides and Mn concentrations Our attempt to incorporate higher Mn content above 20% Mn, resulted in an additional hexagonal CsMnCl 3 phase, along with Cs 4 Pb(Br/Cl) 6 (Supplementary Figure 5 and Supplementary Note 4 ). Table 1 Structural parameters of Cs 4 Pb(Br/Cl) 6 with varying concentration of Mn, calculated using the Rietveld refinement Full size table Phase stabilization of Cs 4 PbX 6 The versatility of the Cs–Pb–X ternary compounds (particularly Cs 4 PbX 6 and CsPbX 3 ) lies in their ability to interconversion via post-synthetic physical and chemical treatments [29] . The post-synthetic conversion of cubic CsPbX 3 to rhombohedral Cs 4 PbX 6 has been demonstrated via amine- and thiol-mediated extraction of PbBr 2 [30] , while the reverse conversion from Cs 4 PbX 6 to CsPbX 3 has been reported by the insertion of PbX 2 , stripping of CsX, excess oleic acid, and by heat treatment (90 to 180 °C) [18] . These post-synthetic conversion mechanisms are inadequate to explain the simultaneous formation of Cs 4 PbX 6 and CsPbX 3 phases, during synthesis. It has been demonstrated that the phase stabilization of perovskite semiconductors could be achieved by controlling the octahedral tilting via partially substituting Pb 2+ with other metal ions. For instance, substitution of smaller Mn 2+ stabilizes the cubic α-CsPbI 3 phase by reducing the octahedral rotation or tilting via a decrease in the bond angle of Pb–I–Pb below 180°, which is along the interconnected neighboring PbX 6 octahedra through the bridging halide ion [31] . In the present case, a similar octahedral tilting (enhanced) results in the phase stabilization of low-symmetry Cs 4 Pb(Br/Cl) 6 upon Mn 2+ incorporation. A decrease in the Pb–X bond length after Mn doping (10% Mn) to 2.950 Å, than undoped Cs 4 Pb(Br/Cl) 6 (2.991 Å), resulted in an enhanced octahedral tilting, preventing the undesired high-symmetry cubic CsPbX 3 phase (Fig. 1c ). Here, the octahedral tilting in the Cs 4 PbX 6 (X = Br/Cl) is described based on the X–Pb–Cs 1 bond angle along c axis of the unit cell, which changes from 54.94° (undoped) to 54.76° upon Mn incorporation. This octahedral tilting would distort the PbX 6 octahedra, which subsequently lowers the symmetry of crystal structure. It is worth mentioning that only two stable compositions exist in the phase diagram of mixed CsX-PbX 2 , under Cs-rich or Pb-deficient conditions viz., low-symmetry rhombohedral Cs 4 PbX 6 and high-symmetry cubic CsPbX 3 [32] . Therefore, enhanced octahedral tilting upon Mn substitution, result in the formation of only possible low-symmetry Cs 4 PbX 6 phase; at the same time, destabilizing the cubic CsPbX 3 phase under Cs-rich condition. This phase stabilization of 0D Cs 4 PbX 6 via Mn substitution, might favor deeper investigation to their unexplored and intriguing properties. Electronic structure The changes in the electronic structure namely bonding nature and electron density distribution in the Cs 4 PbCl 6 were analyzed with Mn incorporation via maximum entropy method (MEM) using XRD results. In the Cs 4 PbCl 6 , the electron density around Pb and Cl is anisotropic and highly resolved with no feature of electron sharing between Pb and Cl, resembling electrostatic attractive/repulsive forces (Fig. 1d ). Upon Mn substitution a significant change in the local charge density around Pb atom was apparent, suggesting that Mn modulates the electronic structure of the 0D Cs 4 PbCl 6 (Fig. 1e, f ). With increasing Mn content, high electron density distribution between Pb and Cl atoms, suggests covalent bonding nature of (Pb/Mn)–Cl bonds (Supplementary Figure 6 ). This also supports the stronger (Pb/Mn)–Cl bonds or shorter bond lengths of Pb–Cl upon Mn doping, as observed from XRD. The change in local electron density after Mn-doping results in the lattice distortion (also evidenced from octahedral tilting, Fig. 1c ) and could lead to electron-phonon (lattice) coupling and formation of polaron [33] . Recently, the formation of polarons in the Cs 4 PbBr 6 has been reported from density functional theory calculation and transient absorption measurements [10] . In the present case, at variance with the undoped Cs 4 PbX 6 , a strong lattice distortion upon Mn incorporation could eventually enhance the electron-phonon coupling, leading to polaron formation. Therefore, it could be concluded that Mn 2+ incorporation modulates the electronic structure and favors the phase stabilization of Cs 4 PbX 6 , preventing the formation of undesirable CsPbX 3 impurity (Fig. 1g ). Though the phase stabilization of Cs 4 PbX 6 were concluded based on XRD results, this technique has its own limitation of insensitivity to detect any minor crystalline phase below 5% [34] . Henceforth, to further support the phase stabilization, optical characterization was exploited owing to its high sensitivity to detect even trace of fluorescent CsPbX 3 impurity. The excitation and photoluminescence (PL) properties of Cs 4 PbX 6 :Mn colloids were presented in Fig. 2 . The undoped Cs 4 Pb(Br/Cl) 6 exhibited broad emission at 432 nm (ranging 415 to 470 nm) under 365 nm excitation (Fig. 2a ). The broad emission arises from the contribution from “D-states” of the host and 3D CsPb(Br/Cl) 3 impurity (443 nm emission, Supplementary Figure 7 ) , where the former dominates the latter. The presence of CsPb(Br/Cl 3 ) impurity was also evident from the broad absorption ranging 360 to 400 nm in the undoped sample (Fig. 2b ). It is to be noted that D-state emission arise from the charge transfer from halide ions of the PbX 6 octahedra to Pb 2+ ion occupying mismatched neighboring Cs + sites, resulting in the creation of Frenkel excitons localized at the vicinity of Pb ions [19] , [35] . Upon Mn incorporation (5% Mn), a narrow emission band at 420 nm was observed, corresponding to the D-state of Cs 4 Pb(Br/Cl) 6 phase, with feeble emission from CsPb(Br/Cl) 3 impurity. The inclusion of chlorine during Mn doping (MnCl 2 precursor) may contribute meagerly to the D-state emission compared to undoped one. Further increase in Mn content (above 10% Mn), eliminated the CsPb(Br/Cl) 3 impurity as evidenced from its negligible absorption (360–400 nm), absorption narrowing, and unaltered D-state emission (Fig. 2a, b ). The above results reaffirm the strong phase stabilization of Cs 4 PbX 6 in presence of Mn, further corroborating the XRD results (Fig. 1a ) [36] , [37] . The additional orange emission at 599 nm, is assigned to the forbidden Mn 2+ d – d transitions [22] , indicating the presence of exchange coupling between charge carriers of Cs 4 Pb(Br/Cl) 6 and Mn 2+ ions. Further, the single-halide Cs 4 PbX 6 analogs were investigated to understand the role of Mn 2+ on the optoelectronic properties and distinguish them from halide effect, which is a limitation in the mixed halides. The undoped Cs 4 PbBr 6 exhibited two UV emission bands and intense green emission (512 nm) arising from Pb 2+ /D-state emission and CsPbBr 3 impurity, respectively (Supplementary Figure 8 and Supplementary Note 5 ). While in the undoped Cs 4 PbCl 6 , the 414 nm emission corresponds to the band-edge emission of CsPbCl 3 impurity [12] and the hump ranging 450 to 480 nm is assigned to the quantum size effect of CsPbCl 3 . Upon Mn incorporation, a new emission at 400 nm arises from the D-state of Cs 4 PbCl 6 , with less contribution from CsPbCl 3 , compared to undoped one, which completely disappeared with higher Mn (20% Mn) content (Supplementary Figure 4 ), reaffirming the phase stabilization of Cs 4 PbX 6 upon Mn incorporation. Fig. 2 Luminescent properties of Mn 2+ -doped Cs 4 PbX 6 . a PL spectra of Mn 2+ -doped Cs 4 PbX 6 colloids were measured under 365 nm excitation, where X = Br/Cl and Cl, with Mn contents denoted as 0% Mn, 5% Mn, 10% Mn, and 20% Mn and the insets shows the respective samples under 365 nm UV lamp. b UV-Vis spectra of Mn 2+ -doped Cs 4 PbX 6 colloids. c PL spectra of Mn 2+ -doped Cs 4 PbX 6 colloids were measured under 290 nm excitation and the insets shows the respective samples under 254 nm UV lamp. The PL spectra presented are the PL intensities corrected using optical density. The asterix mark denote the 3D CsPb(Br/Cl) 3 phases. FE-SEM images of d undoped Cs 4 Pb(Br/Cl) 6 and e Cs 4 Pb(Br/Cl) 6 :10% Mn, and f , g HR-TEM images of Cs 4 Pb(Br/Cl) 6 :10% Mn. A lattice spacing of 0.31 nm corresponding to (131) plane of rhombohedral structure of Cs 4 Pb(Br/Cl) 6 Full size image The undoped and Mn 2+ -doped Cs 4 PbCl 6 displayed blue and pinkish (combination of D-state ‘blue’ and Mn 2+ ‘orange’) emission under 365 nm, respectively (Fig. 2a , inset). The dual UV absorption bands at 218 and 308 nm, are the characteristic features of Cs 4 Pb(Br/Cl) 6 . The band gaps estimated from the absorption maxima are 3.83, 4.02, and 4.25 eV, for Cs 4 PbBr 6 , Cs 4 Pb(Br/Cl) 6, and Cs 4 PbCl 6 , respectively (Supplementary Figure 8a ), which agrees with the earlier reports [18] . It is interesting to note the increase in Cs 4 PbX 6 host emission after Mn doping (Fig. 2a–c ) in both mixed halide and chloride analog, similar to the perovskite nanocrystals [38] . The host emission increment is more prominent in the mixed halide (Br/Cl) analog than pure chloride, which is presumed to the passivation effect of chloride ion, on the pre-existing defects of the host [38] . Therefore, Mn 2+ doping significantly alters the competitive kinetics between the radiative and non-radiative relaxation process of the Cs 4 PbX 6 host. The PL properties were investigated, by exciting at energies higher than band gap of host (290 nm), due to their strong absorption. Mn 2+ -doped (Br/Cl) samples exhibited dual UV emissions at 372 nm and a hump at 324 nm, arising from optical 3 P 0,1,2 → 1 S 0 transitions of Pb 2+ ion [35] , [39] and henceforth denoted as ‘Pb 2+ ion’ emission (Fig. 2c ) . Unlike at 365 nm excitation, the D-state (420 nm) emission of both undoped and Mn 2+ -doped was either absent or buried in the broad 300 to 450 nm spectral range under 290 nm excitation. A similar, broad Pb 2+ emission (354 nm) was observed for Cs 4 PbCl 6 [12] , without the D-state emission, when excited at 290 nm. With Mn doping, an apparent drop in the 3D CsPb(Br/Cl) 3 emission (ranging 430 to 450 nm) further demonstrates the phase stabilization of Cs 4 PbX 6 (Fig. 2c ). In addition, despite the unaltered Pb 2+ emission, an enhanced Mn 2+ emission in the mixed halides, was observed with increasing Mn concentration, due to efficient energy transfer from Pb 2+ to Mn 2+ . The unusual red-shifted emission from 599 to 635 nm for Cs 4 Pb(Br/Cl) 6 :20% Mn sample, is attributed to the formation of Mn-to-Mn pairs at higher Mn concentration, which reduces the 4 T 1 - 6 A 1 energy gap , resulting in the red shift of Mn 2+ emission [40] . Hence, the phase stabilization of Cs 4 PbX 6 (X = Cl, Br/Cl) with Mn incorporation were demonstrated in the chlorine-dominant system (above 60%), through XRD and optical results. The Mn incorporation was also investigated in bromide analog (Cs 4 PbBr 6 ) for monitoring phase stabilization via XRD and PL results (Supplementary Figures 2 and 8 ). With increasing Mn, the green emission (512 nm) of CsPbBr 3 impurity decreased gradually, which completely disappeared above 70% Mn, suggesting the prevention of CsPbBr 3 impurity in presence of Mn, agreeing with the XRD results. However, unlike Br/Cl and Cl analogs, the bromide counterpart necessitates higher Mn 2+ concentration (above 50% Mn) to stabilize the Cs 4 PbBr 6 structure, which is ascribed to the low substitution ratio of Mn 2+ observed in the bromine-dominated Cs–Pb–Br perovskite-like system [41] . In addition, this leads to residual segregation of CsBr, at higher Mn concentration (above 50% Mn). The above results further validate the phase stabilization of zero-dimensional Cs 4 PbX 6 upon Mn incorporation in all the bromine, Br/Cl, and chlorine analogs. The synthesized Cs 4 Pb(Br/Cl) 6 :10% Mn exhibited cubic morphology with particle size ranging between 20 and 40 nm (Fig. 2d–g ) which is much smaller than undoped one (50 to 120 nm). Further increasing the Mn content did not affect the particle size. It is worthy to note that the emission property of Cs 4 PbX 6 host is independent of the particle size due to its intrinsic structural confinement and extremely localized emissive centers (isolated octahedra). However, the dependence of size and morphology of Cs 4 PbX 6 on the length of alkyl chains of amine surfactant were clearly apparent. Unlike long-chain amines (oleylamine), which lead to a narrow particle size distribution in the 26 ± 4 nm range (mixture of spherical, hexagonal, and cubic morphologies) [20] , the use of shorter-chain octylamine in the present work favored a cubic shape with a relatively wide size distribution. Probing the host emissive states The excitation-dependent PL properties of Cs 4 Pb(Br/Cl) 6 were explored to get insight of multiple luminescent states of the host. A range of excitation wavelengths from 280 to 365 nm (4.40 to 3.40 eV) were employed including excitation energies higher than the band gap of Cs 4 Pb(Br/Cl) 6 host (4.00 eV). At higher excitation energies ( λ ex of 280 nm), dominant D-state emission (432 nm) was accompanied by Pb 2+ emission (324 and 375 nm) for undoped Cs 4 Pb(Br/Cl) 6 (Fig. 3a ). It is to be noted that 432 nm emission is denoted here as D-state emission, disregarding the less contribution from CsPb(Br/Cl) 3 impurity (Fig. 2a ), for the ease of emphasizing on dependence of host emissions (Pb 2+ and D-state) with varying excitation energies. As excitation wavelength increased from 280 to 310 nm, the D-state emission gradually decreased, where Pb 2+ emission remains dominant. While above 310 nm excitation, Pb 2+ emission disappeared due to insufficient energy to excite its 3 P 1 levels and only D-state is retained. Upon Mn doping, the D-state emission completely disappeared in the excitation wavelengths ranging, 280 to 310 nm, exhibiting only Pb 2+ emission (Fig. 3b, c ). The absence of D-state emission after Mn 2+ doping is probably due to suppression of charge-transfer process from PbX 6 octahedra to Pb 2+ occupying Cs + site, primarily at high excitation energies (above 4.0 eV), where both Pb 2+ and D-states are excited. Therefore, the presence of Mn 2+ plays a key role in regulating the optical behavior of molecule-like isolated PbX 6 octahedra in Cs 4 PbX 6 nanocrystals. Fig. 3 Probing the host states at the isolated octahedron with Mn 2+ ion. Colloidal PL spectra measured at different excitation wavelengths ranging 280 to 365 nm for the a undoped Cs 4 Pb(Br/Cl) 6 and b Cs 4 Pb(Br/Cl) 6 :5% Mn. c Emission intensities of Pb 2+ and D-state emission with varying excitation energies for the undoped and Mn-doped Cs 4 Pb(Br/Cl) 6 :5% Mn, d excitation spectra of Cs 4 Pb(Br/Cl) 6 :5% Mn colloids by monitoring at 375 nm (Pb 2+ ion), and 420 nm (D-state), e PL intensity ratio of Mn 2+ to the host emission with respect to varying excitation energies, f PL intensity ratio of Mn 2+ to the host states with varying Mn concentration for Cs 4 PbX 6 colloids, where X = (Br/Cl) and Cl, g origin of host emissions namely Pb 2+ and D-state under high excitation energies, without and with Mn doping at high excitation energies. The solid, dashed, and curved arrows are denoted for optical excitation, emission, and energy transfer processes, respectively. h Strength of energy transfer from the host states namely Pb 2+ and D-state to the Mn 2+ emission are depicted. The upward, downward, and curved arrows are denoted for the optical excitation, emission, and energy transfer processes, respectively Full size image The energy transfer and direct excitation of 3 P 1 levels of Pb 2+ (375 nm) and D-states (420 nm), were explored from excitation spectrum of 5% Mn 2+ -doped Cs 4 Pb(Br/Cl) 6 (Fig. 3d ). The spectrum reveals Pb 2+ ion can be excited at high excitation energies above the band gap of Cs 4 Pb(Br/Cl) 6 host (below 310 nm excitation); while the D-state is excited at lower excitation energies typically below the host band gap, (above 310 nm excitation). A direct excitation of D-state at 280 nm, is also apparent along with Pb 2+ ion [35] . However, the energy transfer between the Pb 2+ and D-state of the host cannot be ruled out for the undoped sample, due to the occurrence of D-state emission in the excitation wavelengths (290 to 310 nm) where only Pb 2+ state is excited, as reported earlier [35] , and is consistent with Cs 4 PbX 6 solids (Supplementary Figure 9 and Supplementary Note 6 ). Moreover, Mn 2+ emission is well-known to be sensitized by the host via energy transfer, where Pb 2+ and D-state sensitizes at high and low excitation energies, respectively. Therefore, Mn 2+ emission at varying excitation energies is determined from the absorption of the corresponding host state and efficiency of energy transfer from host states. The Mn 2+ emission relative to the total host emission (i.e., Pb 2+ + D-state) was the highest at 280 nm, attributing to the efficient energy transfer from the Pb 2+ state, which then gradually decreased at lower excitation energies, apart from 320 nm (Fig. 3e ). Although the direct excitation of both Pb 2+ and D-states is possible at 280 nm, Mn 2+ is sensitized only through Pb 2+ state, owing to the suppression of D-state in presence of Mn. The, dominant Mn 2+ emission at 320 nm excitation, ascribed to the Mn 2+ sensitization from both D-state and partially from Pb 2+ ion. In addition, energy transfer from Pb 2+ ion to Mn 2+ was more efficient than from D-state (Fig. 3f , Supplementary Figure 10 , and Supplementary Note 7 ). Moreover, the presence of Mn 2+ considerably suppresses the D-state emission by blocking the charge-transfer process from isolated octahedra to the D-state, especially at high excitation energies (about 4.3 eV, 280 nm excitation), where both the D-state and Pb 2+ could be directly excited (Fig. 3g ). This may be caused by the weak coupling between electronically decoupled (Pb/Mn)X 6 octahedra and D-state (Pb 2+ at Cs site) which deteriorates the charge transfer between them, due to strong Mn–Cl bond formation. The sensitization of Mn 2+ is predominantly occurs from Pb 2+ than the D-state, due to larger energy difference between Mn 2+ and Pb 2+ states (Fig. 3h ). Moreover, the efficient energy transfer to Mn 2+ dopant in the wide band gap host, due to large energy difference between host and Mn 2+ levels, is well documented [38] . The above results demonstrate that the Mn 2+ incorporation significantly affects the optical properties of host state in Cs 4 PbX 6 nanocrystals. Luminescence efficiency The potential application of perovskite-like Cs 4 PbX 6 as emitting layer in color-converting devices has been explored in colloidal and solid forms (thin films and powders) [16] and is expected to have high conversion efficiency similar to other color converter viz. phosphor [42] . High PL QY has been reported in perovskite colloids by employing ligands to stabilize the nanocrystals [1] , [43] , and thin films (solids) of micron-sized grains [44] , [45] . Here, although PL QY of undoped Cs 4 Pb(Br/Cl) 6 nanocrystal is low (5%), the overall QY substantially increased to 32% upon Mn 2+ doping, under 365 nm excitation (Table 2 , Supplementary Figure 11a , and Supplementary Note 8 ). Highest PL QY of 29% was obtained for Cs 4 Pb(Br/Cl) 6 :10% Mn and Cs 4 PbCl 6 :10% Mn (Table 2 ), which is among the best values reported for Mn 2+ emission (Supplementary Table 8 ) [46] . In addition, Mn 2+ luminescence was the highest at lower (365 nm) and higher excitation energy (290 nm), for Cs 4 Pb(Br/Cl) 6 and Cs 4 PbCl 6 , respectively, due to their suitable band gaps (determined by halide species), enabling efficient energy transfer to Mn 2+ . The overall superior PL QY of Mn 2+ -doped Cs 4 PbX 6 colloids (X = Br/Cl, Cl) is attributed to the spatially confined zero-dimensional structure, and presence of dopant at the isolated octahedra favoring enhanced dopant emission through the localized excitons and high exciton binding energy (Supplementary Figure 11b to 11e ). The reported exciton binding energies of Cs 4 PbBr 6 and Cs 4 PbCl 6 are 353 [3] and 153 eV [47] , respectively, compared to CsPbBr 3 (19 to 62 meV) and CsPbCl 3 (72 meV) [48] , [49] , [50] . These results suggest that the high luminescent Cs 4 PbX 6 nanocrystals doped with Mn 2+ could represent promising emitting materials for efficient solid-state lighting applications. Table 2 PL quantum yield of the Cs 4 PbX 6 colloids in n-octane medium Full size table In the Cs 4 PbX 6 solids, a similar low PL QY was observed for undoped sample, but the overall PL QY increased markedly upon Mn doping in both mixed halide and chloride samples (Supplementary Figure 11e ). PL QY of 21% was obtained for Mn 2+ emission in Cs 4 PbCl 6 solids, under 290 nm excitation (Supplementary Table 9 ). The bright orange emission of Mn 2+ -doped Cs 4 PbX 6 in their solid form, is a unique feature among Mn 2+ -doped perovskite solids (Fig. 4c ). This remarkable PL QY and retention of dopant emission in solid form is the attributes of spatial confinement of low-dimensional Cs 4 PbX 6 induced by isolated octahedra, eventually favoring a stable dopant emission in solids. Fig. 4 Lifetime of Mn 2+ -doped Cs 4 PbX 6 . Time-resolved PL spectra of Cs 4 Pb(Br/Cl) 6 colloids excited at 375 nm and monitoring the D-state and Mn 2+ emission at a 420 and b 600 nm, respectively. c Images of Cs 4 PbX 6 perovskite solids under 254 and 365 nm UV lamp, which are denoted by their respective halides and Mn concentrations Full size image To further elucidate the emission properties of Cs 4 PbX 6 host and Mn 2+ , time-resolved PL results were performed by monitoring the D-state (420 nm) and Mn 2+ emission (600 nm), exciting at 375 nm (Fig. 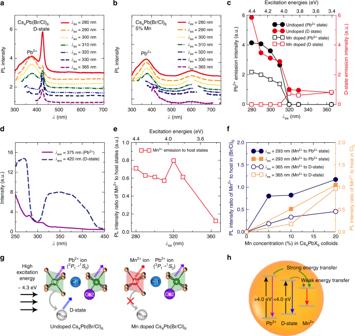4a, b , Supplementary Figures 12 to 14 , and Supplementary Note 9 ). A nominal decrease in the average lifetime of D-state emission in Cs 4 PbX 6 (X = Br/Cl and Cl) was observed with increasing Mn content (Supplementary Figure 13 ). Fig. 3 Probing the host states at the isolated octahedron with Mn2+ion. Colloidal PL spectra measured at different excitation wavelengths ranging 280 to 365 nm for theaundoped Cs4Pb(Br/Cl)6andbCs4Pb(Br/Cl)6:5% Mn.cEmission intensities of Pb2+and D-state emission with varying excitation energies for the undoped and Mn-doped Cs4Pb(Br/Cl)6:5% Mn,dexcitation spectra of Cs4Pb(Br/Cl)6:5% Mn colloids by monitoring at 375 nm (Pb2+ion), and 420 nm (D-state),ePL intensity ratio of Mn2+to the host emission with respect to varying excitation energies,fPL intensity ratio of Mn2+to the host states with varying Mn concentration for Cs4PbX6colloids, where X = (Br/Cl) and Cl,gorigin of host emissions namely Pb2+and D-state under high excitation energies, without and with Mn doping at high excitation energies. The solid, dashed, and curved arrows are denoted for optical excitation, emission, and energy transfer processes, respectively.hStrength of energy transfer from the host states namely Pb2+and D-state to the Mn2+emission are depicted. The upward, downward, and curved arrows are denoted for the optical excitation, emission, and energy transfer processes, respectively For instance, the average lifetime of D-state decreased from 1.08 ns (undoped) to 0.82 ns (20% Mn), corroborating the Mn 2+ sensitization by the Cs 4 Pb(Br / Cl) 6 host (Table 3 ). A long lifetime was obtained for the Mn 2+ emission in Cs 4 Pb(Br/Cl) 6 and Cs 4 PbCl 6 of 1.20 ms and 1.39 ms, respectively (Fig. 4b and Supplementary Figure 13b ). The lifetime of D-states of Cs 4 Pb(Br/Cl) 6 converged with three components namely 3.7 (slow), 2.6, and 0.40 ns (last two combined is fast), similar to the previous report [3] . The first slow (radiative) component is assigned to D-state emission and the fast (non-radiative) component to the energy transfer process to Mn 2+ . A rise in the contribution of slow component with increasing Mn 2+ content, agrees with the increase in D-state emission (Supplementary Figure 12 ). This suggests that the inclusion of chlorine species with Mn-doping (MnCl 2 precursor), passivates the pre-existing defects in the Cs 4 Pb(Br/Cl) 6 host, resulting to an enhanced host PL efficiency [38] . Hence, the passivation effect of chlorine in the Cs 4 Pb(Br/Cl) 6 , would contribute greatly to the PL efficiency of D-state rather than energy transfer to Mn 2+ at 375 nm excitation. On the contrary, superior contribution of fast component in Cs 4 PbCl 6 , illustrates the dominant energy transfer from D-state to Mn 2+ (Supplementary Figures 13 and 14 ) at 375 nm excitation. The chloride passivation effect in the Cs 4 PbCl 6 may be negligible as chloride content remain unchanged with increasing dopant concentration. Therefore, the D-state emission in mixed halide Cs 4 Pb(Br/Cl) 6 , is predominated by the passivation effect of chlorine over energy transfer to Mn 2+ , while in the Cs 4 PbCl 6 , energy transfer to Mn 2+ dominated over passivation effect. Table 3 Average lifetime of D-state emission of Cs 4 Pb(Br/Cl) 6 and Cs 4 PbCl 6 monitored at 420 nm and 400 nm, respectively Full size table The mechanism of energy transfer from host states (Pb 2+ and D-state) to Mn 2+ in the mixed halide perovskite is further illustrated in the Fig. 5 . The high PL QY of Mn 2+ -doped Cs 4 PbX 6 is the attributes of structure-induced quantum confinement with high exciton binding energy favoring enhanced emission, compared to 3D CsPbX 3 perovskite (Fig. 5a ). The superior PL QY of Mn 2+ -doped Cs 4 Pb(Br/Cl) 6 and Cs 4 PbCl 6 were observed at low (365 nm) and high excitation energy (290 nm), due to high absorption in their respective band gaps arising from halide identity. The Pb 2+ ions are excited at high excitation energies (above 4.0 eV), leading to 375 nm emission, while D-states are excited at low excitation energies (below 4.0 eV), and both these states eventually generate Mn 2+ emission through energy transfer (Fig. 5b ). The presence of Mn 2+ suppresses the charge transfer from isolated octahedra to the D-state, due to the weak coupling with the regular crystal lattice sites particularly at higher excitation energy. The enhanced overall PL QY of Mn 2+ -doped Cs 4 PbX 6 in both colloidal and solid form is attributed to the synergistic effect of structural quantum confinement effect from the isolated octahedra and high exciton binding energies, facilitating dopant emission through enhanced energy transfer process. Fig. 5 Mechanism of energy transfer from host states to Mn 2+ . a Illustration of high exciton binding energy (at above 150 meV) due to the localized excitons formed in the isolated octahedra of 0D Cs 4 PbX 6 (X = Cl, Br/Cl) perovskite, compared to low binding energies (less than 60 meV) of 3D CsPbX 3 perovskite, where filled and hollow circles represent electrons and holes, respectively. b Configurational coordinate representation of Cs 4 Pb(Br/Cl) 6 perovskite depicting Pb 2+ -based ( 3 P 0 , 1 → 1 S 0 transition) and D-state emissions, and their energy transfer to the Mn 2+ energy levels. The long dash and dotted arrows depicts the excitation and energy transfer process leading to emission (solid arrows) Full size image In conclusion, we rationalized the exceptional optical behavior of isolated octahedra in the zero-dimensional cesium lead halide structure by introducing Mn 2+ dopants. Structural, PL, and lifetime results confirmed the incorporation of Mn 2+ in the 0D Cs 4 PbX 6 lattice. The Mn 2+ incorporation stabilized the Cs 4 PbX 6 structure via enhanced octahedral tilting and limited compositional variation of Cs–Pb salts, suppressing the formation of CsPbX 3 impurity phase. The PL QY at a given excitation energy was determined by the energy transfer from the host states to Mn 2+ and band gap of the host. A high PL QY for Mn 2+ emission was achieved in the colloidal (29%) and solid (21%, powder) forms; making the solid form of Cs 4 PbX 6 as a promising emissive layer for light-emitting devices. The enhanced PL QY of the Mn 2+ emission was attributed to the synergistic effect of structure-induced spatial confinement of 0D Cs 4 PbX 6 and electronically decoupled PbX 6 octahedra favoring dopant emission via localized exciton. The present work provides deep insight into the structure and molecular behavior of 0D perovskite-like Cs 4 PbX 6 material and opens an avenue to design low-dimensional perovskites with photo and chemical stability for high-performance optoelectronic applications. Materials All the reagents were used without any purification. Cesium carbonate (Cs 2 CO 3 , 99.999% Kojundo), lead (II) bromide (PbBr 2 , 99%, Sigma-Aldrich), lead (II) chloride (PbCl 2 , 98%, Sigma-Aldrich), manganese (II) bromide (MnBr 2 , 98%, Sigma-Aldrich) manganese (II) chloride tetrahydrate (MnCl 2 .4H 2 O, 99%, Sigma-Aldrich), oleic acid (OA, 90%, Fluka), octylamine (OcA, 97%, Sigma-Aldrich), N,N-dimethylformamide (DMF, 99.8%, Sigma-Aldrich), n-hexane (99.8%, Junsei, Japan), n-octane (90%, Sigma-Aldrich), 1-octadecene (95%, Sigma-Aldrich), hydrochloric acid (37%, Sigma-Aldrich), and hydrobromic acid (48%, Sigma-Aldrich) were employed for the synthesis. Synthesis of undoped and Mn 2+ -doped Cs 4 Pb(Br/Cl) 6 colloids The exact compositions of the synthesized undoped and Mn 2+ -doped Cs 4 Pb(Br/Cl) 6 series are Cs 4 PbBr 2 Cl 4 and Cs 4 Pb 1 – x Mn x Br 2–2 x Cl 4+2 x with x = 0.05 (5% Mn), 0.10 (10% Mn), and 0.20 (20% Mn), respectively. Mn 2+ -doped Cs 4 Pb(Br/Cl) 6 nanocrystals were synthesized by a reverse microemulsion method at room temperature, as reported earlier [20] . PbBr 2 precursor was used as the lead precursor. A simultaneous anion (Cl – ) and cation (Mn 2+ ) inclusion were effected by employing MnCl 2 .4H 2 O precursor for the synthesis of Mn 2+ -doped Cs 4 Pb(Br/Cl) 6 . An optimal concentration of octylamine (OcA) and oleic acid (OA) surfactants were used in facilitating the solubilization of Cs, Pb, and Mn precursors. The mixed MnCl 2 .4H 2 O and PbBr 2 precursors, and the Cs-oleate precursor were synthesized separately. First, a mixture of 2.25 g of Cs 2 CO 3 and 21.5 mL of OA was stirred and degassed at 130 °C, which is further maintained under vacuum for 1 h to generate a yellowish stock of Cs-oleate precursor. Second, 0.2 mL Cs-oleate precursor, 10 mL of n-hexane, 5 mL of OA were loaded into a 50-mL three-neck flask, followed by mild degassing (vacuum) for 5 min and Argon purging for 5 min. Third, a mixture of PbBr 2 and MnCl 2 .4H 2 O (DMF, 1 mL), HCl (38 wt%, 19 μL), 0.10 mL OA, and 0.05 mL OcA was swiftly injected into the flask, under vigorous stirring. Upon stirring for 10 min, white color crystals were formed suggesting the formation of Mn 2+ -doped Cs 4 Pb(Br/Cl) 6. The as-synthesized nanocrystals were collected via centrifugation at 7000 rpm for 5 min followed by dispersion in 2 mL of n-octane for further characterization. The contents of Cs-oleate, HCl, and surfactants (OA, OcA) were maintained the same for varying concentration of Mn precursors. The undoped Cs 4 Pb(Br/Cl) 6 was synthesized following the same procedure, in the absence of MnCl 2 .4H 2 O. A color change from a pale-white to green was observed in 10 min upon the addition of Pb precursor into the Cs-oleate, which is then centrifuged and dispersed in n-octane for further characterization. N-octane was employed as the solvent for the Mn 2+ -doped colloids for its superior dispersibility over hexane and toluene. Synthesis of undoped and Mn 2+ -doped Cs 4 PbX 6 (X = Br, Cl) Cs 4 PbX 6 samples were synthesized using stoichiometric quantity of PbX 2 and HX (15 μL) as the lead and halide precursors along with Cs-oleate, where X = Br, Cl. The limited solubility of PbCl 2 in DMF solvent at room temperature was overcome by warming the contents until it gets dissolved. Mn 2+ -doped Cs 4 PbX 6 samples were synthesized following the same procedure along with manganese precursors of MnCl 2 .4H 2 O and MnBr 2 , for the chloride and bromide analog, respectively. Synthesis of CsPbX 3 (X = Br, Br/Cl, Cl) perovskites CsPbX 3 (X = Br, Br/Cl, Cl) nanocrystals were synthesized as described by Palazon et al. [29] . In a typical synthesis, PbX 2 (0.2 mmol; X = Br, Cl, Br/Cl), 0.47 mL oleic acid, 5.0 mL octadecene, and 0.50 mL oleylamine were loaded in a 25 mL 3-neck flask and dried under vacuum at 100 °C for 15 min. The temperature was raised to 190 °C, after degassing and 0.5 mL of Cs-oleate solution (made from 0.4 g of Cs 2 CO 3 dissolved in 11.75 g of octadecene, and 1.55 g oleic acid at 100 °C under vacuum), which was pre-heated on a hot-plate at 100 °C was swiftly injected. Five seconds after the injection, the nanocrystal solution was quickly cooled to room temperature with an ice bath and by the addition of 5 mL of toluene (at 100 °C). The nanocrystals were collected by centrifugation (2500 rpm/2 min.) and re-dispersed in 5 mL toluene. The composition of (Br/Cl) analog is CsPb(Br 0.4 /Cl 0.6 ) 3 , where a mix of 0.08 mmol of PbBr 2 and 0.12 mmol of PbCl 2 precursor were employed for the synthesis. Synthesis of zero-dimensional Cs 4 PbX 6 solids The as obtained colloidal samples dispersed in n-octane were centrifuged and re-dispersed in tert-butanol and centrifuged at 7000 rpm for 5 min. The samples were then dried at 80 °C overnight to get respective Cs 4 PbX 6 solids. The body color of the zero-dimensional solids were pure white for the Cs 4 PbCl 6 , Cs 4 PbCl 6 :Mn, and Cs 4 Pb(Br/Cl) 6 :Mn , except Cs 4 Pb(Br/Cl) 6 (pale greenish white), and Cs 4 PbBr 6 (bright yellow). Characterization The synthesized zero-dimensional Cs 4 PbX 6 nanocrystals were characterized by powder X-ray diffraction (XRD), X-ray photoelectron spectroscopy (XPS), electron spin resonance spectra (ESR), inductive coupled plasma-optical emission spectroscopy (ICP-OES), field-emission scanning electron microscope (FE-SEM), and high-resolution tunneling electron microscope (HR-TEM). The XRD was performed using a Philips X’Pert diffractometer with Cu Kα radiation, in the range of 10° to 120° with a step size of 0.026° with the synthesized powders. The structural information was derived from Rietveld refinement using the General Structure Analysis System (GSAS) software suite. The VESTA program was used to draw the crystal structure [51] . The phase fractions of multiple phases were estimated using Rietveld refinement of XRD results considering full refinement of crystallographic and instrumental parameters as implemented in the GSAS program suite. The FE-SEM and HR-TEM images were recorded using a Hitachi S-4700 and FEI Tecnai F20 (200 kV), respectively, at Korea Basic Science Institute (KBSI), Gwangju, South Korea. The sample for TEM measurements were prepared by dispersing the nanocrystals in the ethanol medium. It is to be noted that the undoped and Mn 2+ -doped Cs 4 PbX 6 perovskite were unstable upon exposure to high-energy electron beam and tend to damage within short period of time. XPS was performed on the powder samples using VG Multilab 2000 instruments to identify the chemical state of the elements on the sample surface (below 10 nm), employing Al as the target anode for the X-ray generation. The energy of the X-ray photon (Al Kα) is 1480 eV with a line width of 0.5 eV. The chemical compositions of the synthesized samples were analyzed using ICP-OES (Perkin-Elmer, OPTIMA 8300), at KBSI, Gwangju, South Korea. ESR measurement was carried out using JEOL JES-FA200 with an X-band microwave frequency of 9.17 GHz, with sample dispersion in n-octane. The liquid samples were taken in an ESR tube and frozen in liquid nitrogen at 173 K. All the spectra were recorded using the following ESR parameters: microwave power, 1 mW; modulation amplitude, 0.2 mT; modulation frequency, 100 kHz; and sweep time, 120 s. Photoluminescence was measured using a Hitachi F-4500 fluorescence spectrophotometer over the wavelength range of 200 to 750 nm, using n-octane dispersions in a 1×1 cm quartz cuvette. UV-vis spectra were obtained using Optizen POP UV/Vis spectrophotometer. The lifetime was measured using a time-correlated single photon counting (TCSPC) system on FL920 Edinburgh instruments at Korean Advance Institute of Science and Technology (KAIST), South Korea. Pulsed laser irradiation with 300 nm was used as the excitation source. Internal quantum efficiency was measured with 365 and 290 nm excitation using a xenon laser (Hamamatsu C9920-02) at the Korea Photonics Technology Institute (KOPTI), South Korea. Time-resolved photoluminescence measurement for Mn 2+ (600 nm) and D-state emission (420 nm for Cs 4 Pb(Br/Cl) 6 and 400 nm for Cs 4 PbCl 6 ) was carried out using single-mode pulsed diode laser as the excitation source ( λ max = 375 nm) at Korea Basic Science Institute (KBSI), Daegu Center, South Korea.